A Nodal-independent and tissue-intrinsic mechanism controls heart-looping chirality Breaking left–right symmetry in bilateria is a major event during embryo development that is required for asymmetric organ position, directional organ looping and lateralized organ function in the adult. Asymmetric expression of Nodal-related genes is hypothesized to be the driving force behind regulation of organ laterality. Here we identify a Nodal-independent mechanism that drives asymmetric heart looping in zebrafish embryos. In a unique mutant defective for the Nodal-related southpaw gene, preferential dextral looping in the heart is maintained, whereas gut and brain asymmetries are randomized. As genetic and pharmacological inhibition of Nodal signalling does not abolish heart asymmetry, a yet undiscovered mechanism controls heart chirality. This mechanism is tissue intrinsic, as explanted hearts maintain ex vivo retain chiral looping behaviour and require actin polymerization and myosin II activity. We find that Nodal signalling regulates actin gene expression, supporting a model in which Nodal signalling amplifies this tissue-intrinsic mechanism of heart looping. Although vertebrates appear externally symmetrical, asymmetries exist within the body cavity. To date, many studies have sought to understand the origins of left–right asymmetry determination in a variety of organisms. Embryonic asymmetric expression of Nodal-related genes is evolutionarily conserved and has been described in a large number of organisms, from snails and sea urchins to chickens and mice [1] , [2] , [3] , [4] , [5] . Knockdown experiments performed in a range of vertebrates have led to a model, wherein this conserved asymmetric Nodal expression is hypothesized to be the driving force behind regulation of organ laterality [1] , [2] , [6] , [7] , [8] . However, these studies have been hampered because of an early requirement for Nodal signalling in primitive streak formation and mesoderm specification [9] . In zebrafish, three homologues of Nodal have been reported— cyclops (cyc), squint (sqt) and southpaw (spaw) [10] , [11] . Although cyc and sqt are expressed during gastrulation and are required for mesendoderm specification, spaw is expressed around the Kupffers vesicle and in the left lateral plate mesoderm (LPM) during somitogenesis stages [10] , [11] . Morpholino oligonucleotide-mediated knockdown of spaw results in loss of asymmetric gene expression and disruption of organ laterality, demonstrating a role for spaw in the regulation of organ asymmetry [11] . Here we present the first described spaw mutant. We show that although intestinal and brain laterality is randomized in spaw mutants, the heart exhibits a previously undescribed preferential looping direction, with the majority of hearts looping in the correct orientation. Genetic and pharmacological inhibition of Nodal signalling demonstrates that this directional bias is independent of Nodal activity. We further show through compound mutant analyses that this directional bias is partly dependent on fluid flow in the Kupffer’s vesicle (KV). Using an ex-vivo heart culture system, we demonstrate that dextral heart looping is a Nodal-independent and tissue-intrinsic process, requiring actomyosin activity. Finally, we show that Nodal signalling regulates actin gene expression, and suggest that asymmetric Nodal signalling may enhance a cytoskeleton-based tissue-intrinsic mechanism of heart looping. The straightforward mutation affects organ laterality The straightforward (sfw) mutant was identified in a forward genetic screen for mutants with organ laterality defects [12] . Whereas the heart in wild-type embryos is positioned asymmetrically under the left eye at 28 h post fertilization (hpf), sfw mutants exhibit a midline heart at 28 hpf ( Fig. 1a,b ) accompanied by no other morphological defects ( Fig. 1c ). Surprisingly, the sfw mutant phenotype displays an uncoupling of cardiac positioning and cardiac looping events; although the initial cardiac tube position (at 28 hpf) is strongly affected in the sfw mutant embryos, cardiac looping (at 48 hpf) is only mildly affected. Analysis of heart laterality at 48 hpf demonstrated that directional looping occurs in 93% of the sfw mutant embryos. Interestingly, in 70% of sfw mutant embryos cardiac looping occurs in the correct dextral direction (d-loop; Fig. 1d , n =796). Expression analysis of marker genes for the atrioventricular canal, working myocardium, endocardium and valves revealed no other cardiac defects in sfw mutant embryos ( Supplementary Fig. S1 ). Interestingly, analysis of endodermal organ positioning in sfw mutants revealed a randomization of digestive system laterality ( Fig. 1e , n =796). In addition, we analysed the left–right asymmetry in the brain by assessing the expression of leftover (lov) , which is expressed in the left habenula of wild-type embryos at 3 days post fertilization (dpf) [13] , and observed a randomization of lov expression in sfw mutants ( Fig. 1f ; n =126). 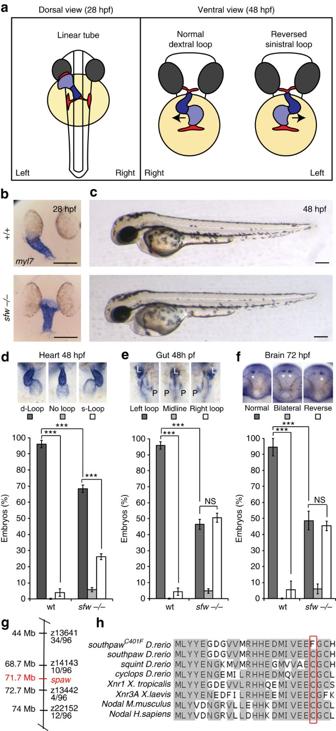Figure 1: Thesfwmutant displays heterotaxia due to loss ofSpawactivity. (a) Schematic depicting cardiac asymmetries observed during zebrafish development. At 28 hpf, the heart is a linear tube positioned under the left eye, which normally undergoes dextral looping by 48 hpf. (b) Analysis of heart position at 28 hpf byin situanalysis ofmyl7expression, dorsal views, anterior to top. (c) Bright-field images of wild-type (wt) andsfwmutant embryos at 48 hpf. (d) Quantification of heart-looping direction at 48 hpf in wt andsfwmutant embryos. Heart is highlighted bymyl7expression. (e) Quantification of digestive system laterality at 48 hpf in wt embryos andsfwmutants, usingfoxA3 in situhybridization to visualize the digestive tract. (f) Quantification of habenulae laterality in wt andsfwmutant embryos at 4 dpf bylov in situhybridization. (d–f) Error bars indicate s.e.m. Significance determined by Student’st-test indicated by asterisks: *P<0.05, **P<0.01, ***P<0.005. (d,e) On the basis of 25 biological replicates (total embryo number=796), (f) based on 3 biological replicates (total embryo number 126). L, liver; P, pancreas; asterisks denote position oflovexpression in the brain. (g) Thesfwmutation was mapped to linkage group 5. x/96 denotes number of recombinants in 96 meioses. Genomic position is noted in Mb. (h) Amino acid alignment of Nodal-related genes in zebrafish,Xenopus, mouse and human. The mutated cysteine residue is highlighted by the red box and is conserved in all Nodals. Scale bars, 100 μM (b,c). Figure 1: The sfw mutant displays heterotaxia due to loss of Spaw activity. ( a ) Schematic depicting cardiac asymmetries observed during zebrafish development. At 28 hpf, the heart is a linear tube positioned under the left eye, which normally undergoes dextral looping by 48 hpf. ( b ) Analysis of heart position at 28 hpf by in situ analysis of myl7 expression, dorsal views, anterior to top. ( c ) Bright-field images of wild-type (wt) and sfw mutant embryos at 48 hpf. ( d ) Quantification of heart-looping direction at 48 hpf in wt and sfw mutant embryos. Heart is highlighted by myl7 expression. ( e ) Quantification of digestive system laterality at 48 hpf in wt embryos and sfw mutants, using foxA3 in situ hybridization to visualize the digestive tract. ( f ) Quantification of habenulae laterality in wt and sfw mutant embryos at 4 dpf by lov in situ hybridization. ( d – f ) Error bars indicate s.e.m. Significance determined by Student’s t -test indicated by asterisks: * P <0.05, ** P <0.01, *** P <0.005. ( d , e ) On the basis of 25 biological replicates (total embryo number=796), ( f ) based on 3 biological replicates (total embryo number 126). L, liver; P, pancreas; asterisks denote position of lov expression in the brain. ( g ) The sfw mutation was mapped to linkage group 5. x/96 denotes number of recombinants in 96 meioses. Genomic position is noted in Mb. ( h ) Amino acid alignment of Nodal-related genes in zebrafish, Xenopus , mouse and human. The mutated cysteine residue is highlighted by the red box and is conserved in all Nodals. Scale bars, 100 μM ( b , c ). Full size image To determine whether aberrant left–right patterning was responsible for the observed organ laterality defects, we analysed the expression of known laterality genes. In wild-type embryos, the Nodal-related gene, spaw , is robustly expressed around the KV (the equivalent organ to the node for the zebrafish) and in the left LPM ( Fig. 2e,f ) [11] . We found that although spaw expression was initiated around the KV and in the posterior LPM in sfw mutant embryos at 10 somites (64%, n =149, Fig. 2g ), by 18 hpf (18 somites) spaw expression had not propagated anteriorly in the left LPM of sfw mutants (100%, n =95; Fig. 2h ). Similarly, lefty1 , a Nodal antagonist expressed in the midline of wild-type embryos ( Fig. 2a,b ), was induced but not maintained nor propagated anteriorly in the midline of sfw mutants ( Fig. 2c,d ). Consistent with the loss of spaw expression in the left anterior LPM of sfw mutant embryos, we observed a loss of asymmetric gene expression in the organ anlage, such as lefty2 in the heart, the Nodal-related gene cyclops in the heart and brain, and the Nodal-regulated gene, pitx2 , in the endodermal organ region, ( Fig. 2i–p ). From this analysis, we concluded that the mutation responsible for the sfw phenotype is acting either upstream or at the same level as Nodal signalling. Despite the severe organ laterality defects, which were most often discordant (heterotaxia, Supplementary Table S1 ), sfw mutant embryos were adult viable. Maternal and zygotic sfw mutant embryos derived from in-crosses of sfw mutant adults displayed no additional morphological phenotypes ( Supplementary Fig. S2 ). 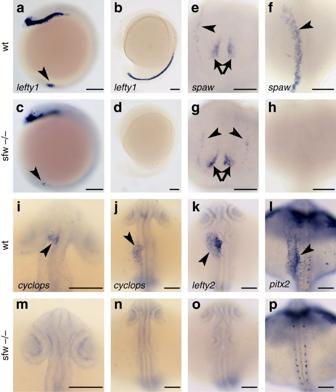Figure 2: Expression of laterality genes is lost insfwmutants. (a–d)In situhybridization analysis oflefty1expression in wild-type (a,b) andsfwmutants (c,d).lefty1is initiated in the caudal notochord in wild-type embryos at 12 hpf (5 somites;a, arrowhead) and its expression expands anteriorly in the midline over the course of somitogenesis (b, 16 hpf, 15 somites). Insfwmutants,lefty1expression is initiated in the midline at 12 hpf (5 somites; c, arrowhead); however, it is not expressed in the midline at 16 hpf (d). (e,f)spawexpression starts around the KV (arrows) and is initiated in the LPM (arrowhead) of wild-type embryos at (14 hpf, 10 somites) (e) and propagates anteriorly during somitogenesis (16 hpf, 15 somites;f, arrowhead). Insfwmutants,spawexpression is initiated around the KV (arrows) and in the posterior LPM (arrowheads) at 14 hpf (g); however,spawexpression does not spread to anterior parts of the LPM later during somitogenesis (h). (i,j)cyclopsis expressed in the left diencephalon (i) and left heart field (j) in wild-type embryos at 21 hpf (23 somites), but is absent from both domains insfwmutant embryos (m,n). (k,l) Wild-type embryos expresslefty2in the left heart field (k) andpitx2in the left LPM (l) at 22 hpf (25 somites); however, expression of bothlefty2in the heart andpitx2in the left LPM is absent insfwmutant embryos (o,p). Scale bars, 100 μM. Figure 2: Expression of laterality genes is lost in sfw mutants. ( a – d ) In situ hybridization analysis of lefty1 expression in wild-type ( a , b ) and sfw mutants ( c , d ). lefty1 is initiated in the caudal notochord in wild-type embryos at 12 hpf (5 somites; a , arrowhead) and its expression expands anteriorly in the midline over the course of somitogenesis ( b , 16 hpf, 15 somites). In sfw mutants, lefty1 expression is initiated in the midline at 12 hpf (5 somites; c, arrowhead); however, it is not expressed in the midline at 16 hpf ( d ). ( e , f ) spaw expression starts around the KV (arrows) and is initiated in the LPM (arrowhead) of wild-type embryos at (14 hpf, 10 somites) ( e ) and propagates anteriorly during somitogenesis (16 hpf, 15 somites; f , arrowhead). In sfw mutants, spaw expression is initiated around the KV (arrows) and in the posterior LPM (arrowheads) at 14 hpf ( g ); however, spaw expression does not spread to anterior parts of the LPM later during somitogenesis ( h ). ( i , j ) cyclops is expressed in the left diencephalon ( i ) and left heart field ( j ) in wild-type embryos at 21 hpf (23 somites), but is absent from both domains in sfw mutant embryos ( m , n ). ( k , l ) Wild-type embryos express lefty2 in the left heart field ( k ) and pitx2 in the left LPM (l) at 22 hpf (25 somites); however, expression of both lefty2 in the heart and pitx2 in the left LPM is absent in sfw mutant embryos ( o , p ). Scale bars, 100 μM. Full size image To determine the position of the mutation underlying the sfw mutant phenotype, we undertook a positional cloning approach. Bulked segregant analysis placed the mutation onto linkage group 5, between markers z13641 and z22152. Fine mapping with simple sequence length polymorphism (SSLP) markers narrowed the region down to a 4-Mb region, including the spaw gene locus ( Fig. 1g ). Sequencing of the entire spaw coding sequence in sfw mutants revealed a single base-pair change that always cosegregated with the sfw mutant phenotype ( Supplementary Fig. S3 ). The identified variant causes a substitution of a conserved cysteine with a phenylalanine at residue 401 of the carboxy terminus of the mature transforming growth factor-β domain ( Fig. 1h ). Although knockdown of Spaw using antisense morpholino oligonucleotides has been shown to result in disrupted organ laterality [11] , we wished to confirm that the uncoupling of cardiac tube position and cardiac looping observed in sfw mutant embryos was due to loss of Spaw function. Analysis of cardiac tube position and cardiac looping in embryos injected with spaw morpholino revealed that although >90% of cardiac tubes remained midline, normal dextral heart looping was observed in a majority of spaw morpholino-injected embryos as was observed for sfw mutant embryos ( Fig. 1 and Supplementary Fig. S3 ). To confirm that the Nodal pathway was disrupted in sfw mutants, we implanted beads soaked in recombinant Nodal protein into the left side of the embryos at the cardiac disc stage before the onset of cardiac tube formation. Implantation of a Nodal bead into sfw mutant embryo completely rescued asymmetric heart tube position when compared with non-implanted controls, demonstrating that the Nodal pathway is indeed disturbed in sfw mutants ( Supplementary Fig. S3 ). To address whether the identified variant affected Spaw function, we injected wild-type spaw and sfw–spaw RNA into embryos and scored for dorsalization due to ectopic Nodal activity [14] , [15] . Overexpression of wild-type spaw and sfw–spaw RNA demonstrated that the C401F variation results in a complete loss of function of Spaw activity ( Supplementary Fig. S3 ). Preferred dextral looping is independent of Nodal signalling As preferred dextral heart looping was maintained in sfw mutants, we wanted to exclude that this resulted from Nodal activity from other Nodal-related proteins such as Cyclops and Squint [10] . We therefore blocked Nodal signalling in sfw mutants using the chemical SB431542 that inhibits the Nodal receptor, Alk7 (ref. 16 ), or by temporally controlled overexpression of the Nodal antagonist, lefty1 ( Supplementary Fig. S4 ). To confirm that application of SB431542 or overexpression of lefty1 -blocked Nodal signalling, we used both techniques at blastula stages and assessed mesoderm formation at 24 hpf, or applied these techniques at the onset of somitogenesis and assessed spaw expression in the LPM at 20 somites. We found that employing both techniques at blastula stages efficiently disrupted formation of mesodermal structures, and that application at the onset of somitogenesis completely abrogated spaw expression, confirming that both techniques effectively block Nodal signalling ( Supplementary Fig. S4 ). We therefore applied SB431542 to wild-type and sfw mutant embryos at 10 hpf, or overexpressed lefty1 in wild-type and sfw mutant embryos at either 10 hpf or 13 hpf, and assessed cardiac-looping direction at 50 hpf. Under all conditions, we still observed preferred dextral heart looping ( Fig. 3a,b and Supplementary Table S2 ). Furthermore, reverse transcription–PCR (RT–PCR) analysis of expression levels of the Nodal homologues cyc and sqt at stages relevant to heart lateralization (13–28 hpf) in wild-type and sfw mutant embryos demonstrated an absence of these genes in sfw mutants ( Supplementary Fig. S4 ), together supporting a model in which d-looping in the absence of Nodal signalling is controlled by an alternative mechanism. 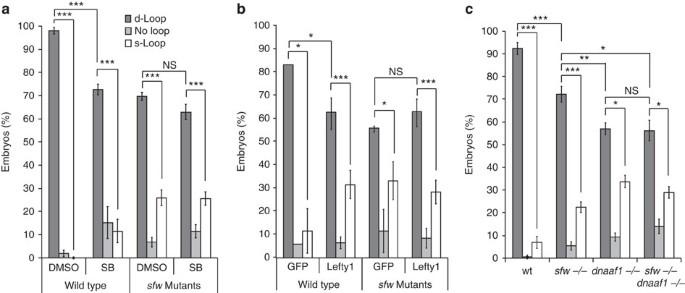Figure 3: Dextral looping bias insfwmutants occurs independently of Nodal activity or KV function. (a) Analysis of looping direction in wild-type (wt) embryos orsfwmutants treated with the Nodal inhibitor SB431542. Wild-type embryos treated with SB431542 show a significant reduction in the number of d-looped hearts when compared with dimethyl sulphoxide (DMSO)-treated controls. However, no significant reduction in the number of d-looped hearts is observed insfwmutant embryos treated with SB431542 when compared with DMSO-treated controls;n=7 clutches of embryos. (b) Analysis of looping direction in wt embryos andsfwmutants, injected with either a uas:gfpcontrol or injected with uas:lft1and heat-shocked at 14 hpf (8–10 somite stage). Wild-type embryos overexpressinguas:lft1showed a significant reduction in the number of d-looped hearts when compared withuas:gfp-injected controls. No significant reduction in the number of d-looped hearts was observed insfwmutants injected with uas:lft1when compared withuas:gfp-injected controls.uas:gfpdatan=4 clutches of embryos,uas:lefty1datan=7. (c) Analysis of looping direction in wt embryos,sfwmutants,dnaaf1mutants andsfw/dnaaf1double mutants.sfwmutants show a significant reduction in the number of d-looped hearts when compared with wild-type embryos.Dnaaf1mutants show a significant reduction in the number of d-looped hearts when compared with eithersfwmutants or wild-type embryos.sfw/dnaaf1double-mutant embryos show a significant reduction in the number of d-looped hearts when compared withsfwmutants or wild-type embryos; however, there is no significant reduction when compared withdnaaf1single mutants.Sfwmutants,dnaaf1mutants andsfw/dnaaf1double mutants all have significantly more dextral looped hearts than sinistral or non-looped hearts;n=10 clutches of embryos. (a–c) Error bars indicate s.e.m. Significance determined by Student’st-test indicated by asterisks: *P<0.05, **P<0.01, ***P<0.005. Figure 3: Dextral looping bias in sfw mutants occurs independently of Nodal activity or KV function. ( a ) Analysis of looping direction in wild-type (wt) embryos or sfw mutants treated with the Nodal inhibitor SB431542. Wild-type embryos treated with SB431542 show a significant reduction in the number of d-looped hearts when compared with dimethyl sulphoxide (DMSO)-treated controls. However, no significant reduction in the number of d-looped hearts is observed in sfw mutant embryos treated with SB431542 when compared with DMSO-treated controls; n =7 clutches of embryos. ( b ) Analysis of looping direction in wt embryos and sfw mutants, injected with either a uas :gfp control or injected with uas :lft1 and heat-shocked at 14 hpf (8–10 somite stage). Wild-type embryos overexpressing uas:lft1 showed a significant reduction in the number of d-looped hearts when compared with uas:gfp -injected controls. No significant reduction in the number of d-looped hearts was observed in sfw mutants injected with uas :lft1 when compared with uas:gfp -injected controls. uas:gfp data n =4 clutches of embryos, uas:lefty1 data n =7. ( c ) Analysis of looping direction in wt embryos, sfw mutants, dnaaf1 mutants and sfw/dnaaf1 double mutants. sfw mutants show a significant reduction in the number of d-looped hearts when compared with wild-type embryos. Dnaaf1 mutants show a significant reduction in the number of d-looped hearts when compared with either sfw mutants or wild-type embryos. sfw / dnaaf1 double-mutant embryos show a significant reduction in the number of d-looped hearts when compared with sfw mutants or wild-type embryos; however, there is no significant reduction when compared with dnaaf1 single mutants. Sfw mutants, dnaaf1 mutants and sfw/dnaaf1 double mutants all have significantly more dextral looped hearts than sinistral or non-looped hearts; n =10 clutches of embryos. ( a – c ) Error bars indicate s.e.m. Significance determined by Student’s t -test indicated by asterisks: * P <0.05, ** P <0.01, *** P <0.005. Full size image Mutant embryos with disrupted cilia-mediated fluid flow in the KV display a wide variety of laterality defects [17] , [18] , [19] . To determine whether the residual cardiac-specific directional bias in sfw mutants is the result of alternative signals under the control of KV function, we analysed heart-looping direction in dnaaf1 mutants with immotile cilia [18] , [19] . Surprisingly, dnaaf1 mutants or sfw/dnaaf1 double-mutant embryos still exhibited a significant preferred dextral heart loop ( Fig. 3c and Supplementary Table S2 ), indicating the existence of a mechanism driving directional heart looping independently of both cilia-induced fluid flow and Nodal signalling. Cardiac disc rotation is dispensable for dextral looping During heart tube formation, the cardiac disc undergoes an asymmetric tissue rearrangement that includes rotation of the cardiac disc and local invagination at the right side. This reorganization results in the left side of the disc, ultimately forming the dorsal face of the heart tube [19] , [20] , [21] . It has been suggested that such rotational events may provide directed torsion in the heart tube, which in turn may drive directional looping [20] , [22] , [23] , [24] , [25] . Previous studies on heart tube formation using spaw knockdown experiments have suggested that in the absence of Nodal, both the direction of cardiac disc rotation and the site of myocardial involution are randomized, resulting in either a leftward or rightward positioning of the cardiac tube [11] , [19] , [21] , [26] . Our observation that the linear heart in sfw mutants is predominantly positioned at the midline and rarely under the left or right eye suggests that the reported randomization in heart position was due to an incomplete spaw knockdown. To determine whether cardiac disc rotation occurs in sfw mutants and whether any degree of rotation is significantly linked to subsequent laterality of heart looping, we imaged heart tube formation in wild-type embryos or sfw mutant embryos between 20 hpf and 24 hpf ( Fig. 4a ), and subsequently raised the embryos to 55 hpf when handedness of cardiac looping could be determined. We tracked individual myocardial cells during linear heart tube formation ( Fig. 4a ) and measured their displacement rates and direction ( Fig. 4b ). We observed that cardiac disc rotation failed to occur in either dextral or sinistral looped hearts of sfw mutant embryos (2.2° and −0.8°, respectively, n =4 for each; Fig. 4c ) and that the overall velocity of cardiomyocytes was significantly slower in sfw mutants ( Supplementary Fig. S5 ). These results demonstrate that cardiac disc rotation is not required for handedness of heart looping. 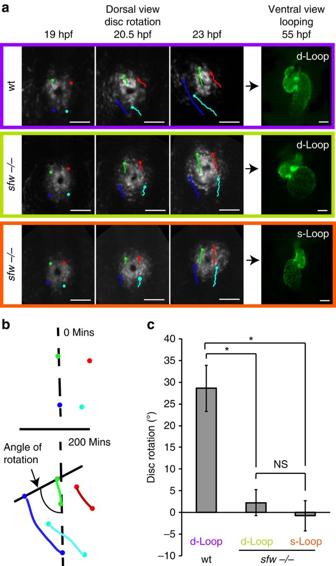Figure 4: Chiral heart looping occurs independently from cardiac disc rotation. (a) Still images (dorsal view, anterior up) from time-lapse movies generated from projected confocal stacks using theTg(myl7:GFP)transgenic line labelling all cardiomyoscytes. Blue, green, red and turquoise traces indicate movement of individual cells in wild-type orsfwmutants embryos between 19.5 hpf and 23 hpf. Ventral view stills indicate direction of heart looping at 55 hpf in time-lapse-imaged embryos. (b) Schematic showing method for analysis of cardiac rotation. (c) Quantification of cardiac disc rotation in wild-type embryos with a d-looped heart,sfwmutants with d-looped heart andsfwmutants with s-looped heart (n=4 for each category). Error bars indicate s.e.m. Significance determined by Student’st-test indicated by asterisks: *P<0.05;n=4 embryos for each category (wild-type, d-loop mutant, s-loop mutant). Scale bars, 50 μM (a). Figure 4: Chiral heart looping occurs independently from cardiac disc rotation. ( a ) Still images (dorsal view, anterior up) from time-lapse movies generated from projected confocal stacks using the Tg(myl7:GFP) transgenic line labelling all cardiomyoscytes. Blue, green, red and turquoise traces indicate movement of individual cells in wild-type or sfw mutants embryos between 19.5 hpf and 23 hpf. Ventral view stills indicate direction of heart looping at 55 hpf in time-lapse-imaged embryos. ( b ) Schematic showing method for analysis of cardiac rotation. ( c ) Quantification of cardiac disc rotation in wild-type embryos with a d-looped heart, sfw mutants with d-looped heart and sfw mutants with s-looped heart ( n =4 for each category). Error bars indicate s.e.m. Significance determined by Student’s t -test indicated by asterisks: * P <0.05; n =4 embryos for each category (wild-type, d-loop mutant, s-loop mutant). Scale bars, 50 μM ( a ). Full size image Heart-intrinsic dextral looping requires actomyosin activity Isolated linear heart tubes from chick and amphibian embryos maintain their ability to form a dextral loop ex vivo [27] , [28] . We therefore hypothesized that in the absence of Nodal signalling, preferential dextral cardiac looping is maintained due to an alternative tissue-intrinsic mechanism. To test this hypothesis, we developed an ex-vivo heart culture system by manually dissecting linear heart tubes from zebrafish embryos at 28 hpf and culturing these in supplemented tissue culture medium ( Fig. 5a ). Indeed, we observed that linear heart tubes of both wild-type embryos and sfw mutant embryos underwent looping after 24 h in culture ( Fig. 5b ). Furthermore, we observed that 79% of explanted wild-type hearts displayed a dextral loop after 24 h in culture ( Supplementary Fig. S6 ). 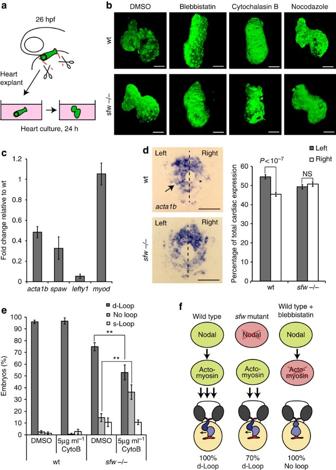Figure 5: Heart looping is a tissue-intrinsic process that requires actomyosin activity. (a) Schematic depicting the heart explant system. Linear heart tubes were dissected fromTg(myl7:GFP)-positive embryos at 26 hpf, placed into culture medium and incubated for 24 h before fixation and imaging. (b) Explanted linear heart tubes of wild-type orsfwmutant embryos were treated with either dimethyl sulphoxide (DMSO), Blebbistatin, Cytochalasin B or Nocodazole duringex vivoculturing for 24 h. (c) Quantitative RT–PCR analysis of relative levels of expression ofacta1b,spaw,lefty1ormyodinsfwmutants compared with wild-type embryos at 21 hpf (23 somites).Acta1b,spawandlefty1expression was downregulated insfwmutant embryos, whereasmyoDexpression was unaffected. Three biological replicates were used and each biological sample was analysed in triplicate. (d) In situ hybridization analysis ofacta1bexpression in wild-type andsfwmutant embryos at 21 hpf. Quantification by image analysis of relative levels of expression between the left and right sides of the cardiac fields revealed that wild-type embryos had elevatedacta1bexpression in the left cardiac field (arrow) compared with the right side (asterisk), whereassfwmutants had no asymmetric elevation ofacta1bexpression. Thirty-six embryos from two biological replicates were analysed. (e) Heart-looping direction in wild-type embryos orsfwmutants treated with either DMSO or 5 μg ml−1Cytochalasin B between 26 hpf and 55 hpf. Treatment of wild-type embryos with Cytochalasin B had no effect on heart-looping direction, whereas treatment ofsfwmutant embryos with Cytochalasin B significantly reduced the number of dextral looped hearts and increased the number of non-looped hearts;n=9 clutches of embryos. (c–e) Error bars indicate s.e.m. Significance determined by Student’st-test indicated by asterisks: **P<0.01. (f) Cartoon illustrating possible regulation of dextral heart looping by Nodal and actomyosin. In a wild-type situation, combined Nodal signalling and actomyosin activity provide a robust mechanism driving dextral heart looping. In the absence of Nodal signalling, actomyosin activity is sufficient to promote preferential dextral heart looping. In the absence of actomyosin activity, Nodal signalling is not sufficient to promote dextral heart looping. Scale bars, 50 μM (b,d). Figure 5: Heart looping is a tissue-intrinsic process that requires actomyosin activity. ( a ) Schematic depicting the heart explant system. Linear heart tubes were dissected from Tg(myl7:GFP) -positive embryos at 26 hpf, placed into culture medium and incubated for 24 h before fixation and imaging. ( b ) Explanted linear heart tubes of wild-type or sfw mutant embryos were treated with either dimethyl sulphoxide (DMSO), Blebbistatin, Cytochalasin B or Nocodazole during ex vivo culturing for 24 h. ( c ) Quantitative RT–PCR analysis of relative levels of expression of acta1b , spaw , lefty1 or myod in sfw mutants compared with wild-type embryos at 21 hpf (23 somites). Acta1b , spaw and lefty1 expression was downregulated in sfw mutant embryos, whereas myoD expression was unaffected. Three biological replicates were used and each biological sample was analysed in triplicate. ( d ) In situ hybridization analysis of acta1b expression in wild-type and sfw mutant embryos at 21 hpf. Quantification by image analysis of relative levels of expression between the left and right sides of the cardiac fields revealed that wild-type embryos had elevated acta1b expression in the left cardiac field (arrow) compared with the right side (asterisk), whereas sfw mutants had no asymmetric elevation of acta1b expression. Thirty-six embryos from two biological replicates were analysed. ( e ) Heart-looping direction in wild-type embryos or sfw mutants treated with either DMSO or 5 μg ml −1 Cytochalasin B between 26 hpf and 55 hpf. Treatment of wild-type embryos with Cytochalasin B had no effect on heart-looping direction, whereas treatment of sfw mutant embryos with Cytochalasin B significantly reduced the number of dextral looped hearts and increased the number of non-looped hearts; n =9 clutches of embryos. ( c – e ) Error bars indicate s.e.m. Significance determined by Student’s t -test indicated by asterisks: ** P <0.01. ( f ) Cartoon illustrating possible regulation of dextral heart looping by Nodal and actomyosin. In a wild-type situation, combined Nodal signalling and actomyosin activity provide a robust mechanism driving dextral heart looping. In the absence of Nodal signalling, actomyosin activity is sufficient to promote preferential dextral heart looping. In the absence of actomyosin activity, Nodal signalling is not sufficient to promote dextral heart looping. Scale bars, 50 μM ( b , d ). Full size image In Drosophila and Caenorhabditis elegans , both of which lack Nodal genes in their genome, laterality is controlled by tissue- and cell-intrinsic mechanisms that require specific components of the cytoskeleton [29] , [30] , [31] , [32] , [33] , [34] . Similarly, cultured mammalian cells show phenotype-specific left–right asymmetry that is controlled by the cells cytoskeleton [33] , [34] . To determine whether the tissue-intrinsic and Nodal-independent mechanism that controls heart looping requires specific components of the cytoskeleton, we treated explants of linear heart tubes with various inhibitors affecting normal cytoskeleton formation. We observed normal heart looping in wild-type and sfw mutant hearts treated with either dimethyl sulphoxide or Nocodazole during the culturing period ( Fig. 5b ), indicating that microtubule formation is dispensable for normal heart looping. However, explanted hearts incubated with either the myosin II inhibitor, Blebbistatin, or the actin polymerization inhibitor, Cytochalasin B, displayed compromised looping and a failure of constriction at the atrioventricular canal ( Fig. 5b ), indicating that both the actin cytoskeleton and its interactions with non-muscle myosin II are specifically required for the tissue-intrinsic cardiac remodelling that underlies heart looping. This requirement for myosin II in cardiac looping was also observed in wild-type embryos and is independent from its role in cardiac contractility, as we found that mutant hearts defective in cardiac contractility displayed normal dextral looping ( Supplementary Fig. S7 ). Nodal signalling regulates actin levels How can two mechanisms (a Nodal-dependent and a Nodal-independent mechanism) efficiently control handedness of heart looping? The asymmetric Nodal expression in the LPM could amplify the heart-intrinsic mechanism that requires actomyosin activity. Indeed, in chick and mouse embryos with asymmetric Nodal activity, messenger RNA of genes encoding cytoskeleton components or their products localize asymmetrically in the heart tube [35] , [36] . Several actin-related genes are expressed in the embryonic zebrafish heart [37] , [38] and RT–PCR analysis revealed that α-actin1b ( acta1b ) was downregulated in sfw mutant embryos before heart looping ( Fig. 5c ). In situ hybridization combined with image analysis revealed that acta1b is expressed asymmetrically in the wild-type heart at 23 somites (21 hpf) before leftward displacement, with elevated expression of acta1b on the left side of the cardiac disc compared with the right side ( Fig. 5d ). This left-sided elevation of acta1b was lost in sfw mutants. If the asymmetric Nodal expression in the LPM amplifies a heart-intrinsic mechanism by elevating actin levels, then hearts of sfw mutant embryos lacking asymmetric Nodal activity should be more prone to perturbations of actin polymerization. Corroborating such a model, we observed that treatment of wild-type embryos with a low concentration of Cytochalasin B had no effect on heart looping, whereas the same treatment efficiently perturbed heart looping in sfw mutants ( Fig. 5e ). We conclude that chiral heart looping is a tissue-intrinsic process that is controlled by both Nodal-dependent and -independent mechanisms. We suggest the following model (shown in Fig. 5f ) to explain our observations. In the presence of asymmetric Nodal signalling, actin polymerization in the heart tissue is elevated and clockwise rotation of the cardiac disc and leftward displacement of the linear heart tube are observed, resulting in robust dextral looping in almost all embryos. In the absence of Nodal signalling, actin levels are reduced (shown in Fig. 5 ), and cardiac rotation and leftward displacement of the heart tube are perturbed (shown in Figs 1 and 4 ). In this situation, directional heart looping is maintained in most embryos due to a tissue-intrinsic mechanism that requires actin polymerization and myosin II activity (shown in Figs 1 and 3 , 4 , 5 ). When actomyosin activity is blocked, even in the presence of asymmetric Nodal signalling, directional heart looping is prevented (shown in Fig. 5 ). Our study provides strong evidence that contrary to current models although Nodal signalling is instructive in promoting correct laterality in the heart, it is not the sole pathway regulating chirality of heart looping. Asymmetric Nodal expression is not only widely conserved between higher vertebrates, but has also been observed in the lower chordates, such as ascidians and lancelets [39] , [40] . Interestingly, although these ancestral organisms exhibit asymmetric embryonic Nodal expression, accompanied by brain and gut asymmetries, no heart asymmetries are observed in the developing embryo [41] , [42] . This suggests that ancestrally the heart did not respond to asymmetric Nodal signalling [43] and it is interesting to speculate that heart asymmetry developed independent of asymmetric Nodal. Supporting this, we demonstrate that chiral looping is intrinsic to the heart tissue itself, even in the absence of Nodal signalling. It is tempting to speculate that regional polarization of cardiomyoctes combined with specific coordinated movement of regionalized cells results in organ-intrinsic heart looping. Corroborating such a mechanism are recent studies demonstrating that various cell lines exhibit intrinsic left–right polarity [33] , [34] , [44] , whereas elegant imaging analyses have demonstrated regionalized cell polarity coordination in the mouse heart during development [45] . Our study demonstrates that subsequent to gastrulation, Nodal signalling is dispensable for directional heart looping. The Nodal-related genes sqt and cyc are expressed early during gastrulation and are required for mesoderm formation—loss of these factors early during development results in an absence of cardiac mesoderm. Therefore, we cannot exclude a very early role for Nodal during mesoderm formation in promoting left–right asymmetries in the heart; however, to date, no left–right asymmetry in Nodal activity during gastrulation stages has been reported. Furthermore, we demonstrate that non-muscle myosin II activity and actin polymerization are essential for cardiac looping. Although asymmetric actin bundles in the right side of the chick heart have been shown to be important for regulating dextral looping [35] , the role of non-muscle myosins in total organ laterality and more specifically in heart laterality is beginning to be uncovered. The unconventional non-muscle myosin MYO31DF is required for correct organ laterality in Drosophila [29] , [30] . Similarly, recent studies in C. elegans and zebrafish suggest that non-muscle myosins are required for symmetry breaking in the early embryo [32] , [46] . Moreover, asymmetric localization of non-muscle myosin II was observed in the cardiac fields before linear heart tube formation in zebrafish and mouse embryos [36] , [47] , and mouse embryos lacking non-muscle myosin II-B exhibit structural cardiac defects that could be related to incomplete heart looping [48] . It is interesting to hypothesize that actomyosin-based cytoskeletal processes may regulate cardiac laterality at a cellular or regional level through asymmetric epithelial morphogenesis. It has been demonstrated that cell-intrinsic laterality is dependent on cytoskeletal components, and that disruption of these components results in loss of directionally biased cellular migration [33] . Furthermore, it has been suggested that polarized actomyosin contractility drives the junctional remodelling required for epithelial morphogenesis [49] . Possibly asymmetric actomyosin contractility in the zebrafish heart drives directional cardiomyocyte migration, resulting in the epithelial remodelling characteristic of heart looping. The mechanism by which such cells acquire polarized actomyosin activity remains unclear, although it is also possible that tissue tension within the heart, driven by addition of cells from the second heart field to the growing heart tube, orients actin localization or myosin recruitment similar to the orientation of tissue polarity by cellular flow in Drosophila axis and wing elongation [50] , [51] . Together, these data support that organ laterality is promoted by cytoskeletal remodelling processes that are conserved between species. Fish lines and husbandry The following zebrafish lines were used: Tg(cmlc2:GFP ) [52] , sfw(Tg:cmlc2:GFP) , TL, dnaaf hu255H (ref. 18 ) and hsp70:gal4 (ref. 53 ). Fish were maintained according to standard laboratory conditions. Animal experiments were approved by the Animal Experimentation Committee (DEC) of the Royal Netherlands Academy of Arts and Sciences. The N-ethyl-N-nitrosourea-mediated mutagenesis screen was performed by mutagenizing ~100 adult male zebrafish by three to five consecutive treatments with 3 mM N-ethyl-N-nitrosourea. The mutagenized males were crossed to wild-type females to generate F1 families. F1 progeny were subsequently outcrossed to wild-type embryos to create ~300 F2 families. The F2 families were incrossed and the F3 progeny screened for cardiac laterality defects at 28–32 hpf. Positional cloning of the sfw mutant The spaw t30973 allele was mapped by standard meiotic mapping using SSLPs. Sequences for the primers used for SSLP mapping can be found in Supplementary Table S3 . The spaw t30973 mutant can be identified using PCR amplification, followed by Eco RI restriction of the PCR product using the following primers: forward primer: 5′-GGACATGATCGTGGAGGAAT-3′ and reverse primer: 5′-TCAGGAGTCGCCACAGTAGA-3′; the primers introduce an Eco RI restriction site into the mutant strand. In situ hybridization Embryos were fixed overnight in 4% paraformaldehyde (PFA) and stored in MeOH. Embryos were rehydrated to PBST (PBS plus 0.1% Tween) and treated with 1 μg ml −1 Proteinase K for between 1 and 20 min depending on the stage. Embryos were rinsed in PBST, post fixed in 4% PFA for 20 min, washed 3 × 5 min in PBST and pre-hybridized for at least 1 h in Hyb-buffer. Riboprobes were diluted in Hyb-buffer supplemented with transfer RNA and heparin, and incubated with embryos overnight at 70 °C. Following probe removal, embryos were washed stepwise from Hyb- to 2 × SSC, and subsequently from 0.2 × SSC to PBST. Embryos were blocked for at least 1 h in PBST supplemented with sheep serum and BSA before being incubated overnight at 4 °C with anti-digoxygenin antibody. Following antibody removal, embryos were washed extensively in PBST before being washed several times in TBST. Nitro-blue tetrazolium/5-bromo-4-chloro-3-inodyl phosphate was diluted in TBST, added to embryos and protected from the light. Once staining had developed, embryos were washed several times in PBST and fixed overnight in 4% PFA. Embryos were cleared in MeOH and mounted in benzylbenzoate:benzylalcohol (2:1) before imaging. Riboprobes were transcribed from linearized template in the presence of 11-UTP. The acta1b in situ was quantified by measuring pixel intensity in the left side and right side of the cardiac disc and was normalized to background levels (using ImageJ software). Total pixel intensity was then determined and the percentage contribution of left or right side to total intensity was calculated. mRNA and DNA microinjections Full-length spaw complementary DNA was cloned into the PCS2+ vector (Addgene). The sfw mutation was introduced into the spaw PCS2+ construct by site-directed mutagenesis using a Quickchange kit (Stratagene). Injection mRNA was transcribed using the SP6 mMessage mMachine kit (Ambion). The spaw morpholino targeting the intron 2–exon 3 splice site (5′-TGGTAGAGCTTCAACAGACTCTGCA-3′) was injected at the one-cell stage at 5 ng (ref. 11 ). Full-length lefty1 open reading frame was amplified from wild-type cDNA. The full-length fragment was cloned into a vector containing 14 × UAS promoter and a polyA tail. Embryos were injected at the one-cell stage with 5 pg of UAS : lft1 and 5 pg of UAS:GFP . Heat-shock experiments were performed by placing embryos in preheated E3 medium at 37 °C for 30 min. Time-lapse analysis Embryos were dechorionated and mounted in 0.25% agarose. Images were acquired using a Leica SP2 confocal microscope and confocal stacks were acquired every 4 min for 4 h. Embryos were subsequently excised from the agarose and raised to 50 hpf. Cells were manually tracked using ImageJ software. Rotation was calculated as an average of angles or rotation from both left and right sides of the heart. A vertical line is drawn between two cells in one side of the heart. A line is drawn between the same cells at the end of the time lapse and the angle between these two lines is taken as a measure of rotation. For velocity analysis, individual cell velocities at each time point during time lapse were calculated in ImageJ, and average velocities for all cells over time in either the anterior or posterior region of the heart were determined. Chemical treatments Embryos were soaked in 100 μM of the Nodal inhibitor SB431542 (Sigma), 25 μM Blebbistatin (Sigma) or 5 μg ml −1 Nocodazole (Sigma) in a final concentration of 1% dimethyl sulphoxide in E3 medium. After timed treatments, embryos were washed 4 × 5 min in fresh E3 medium before fixation. Bead implants Agarose beads (Affigel blue, Biorad) were rinsed twice in PBS and incubated for 1 h at 37 °C with 50 μg ml −1 recombinant mouse Nodal protein (R&D Systems). Embryos at the 15–18 somite stage were mounted in 0.25% agarose and beads were inserted under the left eye using a tungsten needle. Embryos were excised from the agarose and fixed at 28 hpf. Heart explants and drug treatments Hearts were manually dissected from 26 hpf embryos using forceps and placed into supplemented L15 culture medium (15% fetal bovine serum, 0.8 mM CaCl 2 , 50 μg ml −1 penicillin, 0.05 mg ml −1 streptomycin, 0.05 mg ml −1 gentomycin) [54] . Explants were incubated at 28.5 °C for 24 h and fixed in 4% PFA overnight. Explants were treated with Blebbistatin (25 μM, Sigma), Cytochalasin B (5 μg ml −1 , Sigma) or Nocodazole (100 ng ml −1 , Sigma). Explanted hearts were mounted in Vectashield or Mowiol, and imaged using a Leica SPE confocal microscope. Three-dimensional reconstructions were generated using Volocity (Improvision). Quantitative RT–PCR Total RNA was extracted from 19.5 hpf wild-type and sfw mutant embryos. cDNA was generated using the RTIII First Strand kit (Invitrogen). Quantitative PCRs were performed using SYBR Green (BioRad) in a BioRad MyIQ PCR machine. Gene expression levels were normalized to gapdh and ef1a levels. Three biological repeats were used for each genotype and reactions were performed in triplicate. How to cite this article: Noël, E. S. et al. A Nodal-independent and tissue-intrinsic mechanism controls heart-looping chirality. Nat. Commun. 4:2754 doi: 10.1038/ncomms3754 (2013).